Yeast and mammalian autophagosomes exhibit distinct phosphatidylinositol 3-phosphate asymmetries Phosphatidylinositol 3-kinase is indispensable for autophagy but it is not well understood how its product, phosphatidylinositol 3-phosphate (PtdIns(3)P), participates in the biogenesis of autophagic membranes. Here, by using quick-freezing and freeze-fracture replica labelling, which enables determination of the nanoscale distributions of membrane lipids, we show that PtdIns(3)P in yeast autophagosomes is more abundant in the luminal leaflet (the leaflet facing the closed space between the outer and inner autophagosomal membranes) than in the cytoplasmic leaflet. This distribution is drastically different from that of the mammalian autophagosome in which PtdIns(3)P is confined to the cytoplasmic leaflet. In mutant yeast lacking two cytoplasmic phosphatases, ymr1Δ and sjl3Δ , PtdIns(3)P in the autophagosome is equally abundant in the two membrane leaflets, suggesting that the PtdIns(3)P asymmetry in wild-type yeast is generated by unilateral hydrolysis. The observed differences in PtdIns(3)P distribution suggest that autophagy in yeast and mammals may involve substantially different processes. Macroautophagy (hereafter referred to as autophagy) plays important roles in a wide range of physiological phenomena, and dysfunctions in this process are involved in various diseases [1] . In autophagy, portions of the cytoplasm are surrounded by an expanding membrane sac, called the isolation membrane or phagophore, which eventually matures into double-membrane structures called autophagosomes. Autophagosomes fuse with lysosomes (or vacuoles, in yeast and plants), after which the engulfed cytoplasmic contents (as well as the inner of the two autophagosomal membranes) are degraded. Functional analyses of Atg proteins have revealed the details of many aspects of autophagy [2] , but the origin of the autophagosomal membrane has remained an enigma [3] . In yeast, the isolation membrane is thought to originate from the pre-autophagosomal structure (PAS), in which Atg proteins assemble in a hierarchical manner [4] . The PAS is observed as a perivacuolar dot under the fluorescence microscope, but no membranous structure has been identified at that site. In mammals, the PAS has not been identified and the isolation membrane is thought to form from existing organelles [5] , [6] , [7] , [8] . In both yeast and mammals, phosphatidylinositol 3-kinase (PtdIns 3-kinase) activity is indispensable for autophagy [9] , [10] , and its product, phosphatidylinositol 3-phosphate (PtdIns(3)P), is thought to play critical roles in this process. In a previous study using green fluorescent protein (GFP)-tagged biosensors in live cells, PtdIns(3)P was detected in the isolation membrane, where it may promote concentration of PtdIns(3)P-binding proteins on the membrane [11] . As recruitment of PtdIns 3-kinase to the site of isolation membrane formation is one of the first events in autophagy both in yeast and mammals, we speculated that a detailed analysis of PtdIns(3)P distribution might provide clues concerning the origin of the autophagic membrane. However, such an analysis is technically challenging: live imaging using GFP-tagged biosensors has low spatial resolution and may perturb the distributions of target lipids [12] . Furthermore, electron microscopy (EM) using chemically fixed samples is not appropriate, because most membrane lipids are not immobilized by aldehydes [13] . Therefore, we employed the quick-freezing and freeze-fracture replica labelling method (QF-FRL), which enables nanoscale membrane lipid labelling by physically fixing membrane molecules [14] , [15] , [16] . This technical advantage is important for analysis of the autophagosome, in which the double membranes are only narrowly separated. Using the QF-FRL method, we found that PtdIns(3)P exhibits drastically different distributions in yeast and mammalian autophagosomes. Most notably, PtdIns(3)P in the yeast autophagosome is present in the membrane leaflet facing the closed space between the outer and inner autophagosomal membranes, whereas in mammalian autophagosome PtdIns(3)P is confined to the membrane leaflet facing the cytoplasm. This difference in distribution of a key lipid suggests that membrane dynamics in autophagy in yeast and mammals may proceed in fundamentally different ways. Specific labelling of PtdIns(3)P by QF-FRL method To find an appropriate probe for PtdIns(3)P in QF-FRL, we tested several protein domains tagged with glutathione S -transferase (GST), including the FYVE domain of human Hrs and FENS-1, and the PX domain of human p40 phox (ref. 17 ). Using a freeze-fracture replica of liposomes made of 95% phosphatidylcholine and 5% phosphoinositides, we found that the PX domain of p40 phox labelled PtdIns(3)P specifically and most intensely ( Fig. 1a ). The labelling specificity was further confirmed by the observation that a mutant GST-PX R58A that lacks PtdIns(3)P-binding ability [18] yielded virtually no labelling in the PtdIns(3)P liposome replica when used at the same concentration as GST-PX ( Fig. 1a ). 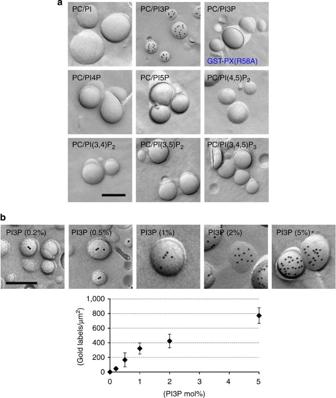Figure 1: QF-FRL of liposomal replicas. (a) QF-FRL of unilamellar liposomes containing 95 mol% of phosphatidylcholine and 5 mol% of a phosphoinositide, labelled with GST-PX. Only liposomes containing PtdIns(3)P were labelled intensely. GST-PXR58A, a PX-domain mutant that does not bind PtdIns(3)P, yielded virtually no labelling in PtdIns(3)P-containing liposomes. Scale bar, 0.2 μm. (b) QF-FRL of unilamellar liposomes containing 0–5 mol % of PtdIns(3)P. Scale bar, 0.2 μm. The labelling density increased roughly in proportion to the PtdIns(3)P content of the liposomes. The experiment was repeated twice and the number of colloidal gold particles per μm2was measured in more than 75 randomly selected liposomes. Values for all concentrations are statistically different from those in the adjacent conditions (for example, 1 versus 2 mol%; mean±s.e.m.; Student’st-test;P<0.05). Figure 1: QF-FRL of liposomal replicas. ( a ) QF-FRL of unilamellar liposomes containing 95 mol% of phosphatidylcholine and 5 mol% of a phosphoinositide, labelled with GST-PX. Only liposomes containing PtdIns(3)P were labelled intensely. GST-PX R58A , a PX-domain mutant that does not bind PtdIns(3)P, yielded virtually no labelling in PtdIns(3)P-containing liposomes. Scale bar, 0.2 μm. ( b ) QF-FRL of unilamellar liposomes containing 0–5 mol % of PtdIns(3)P. Scale bar, 0.2 μm. The labelling density increased roughly in proportion to the PtdIns(3)P content of the liposomes. The experiment was repeated twice and the number of colloidal gold particles per μm 2 was measured in more than 75 randomly selected liposomes. Values for all concentrations are statistically different from those in the adjacent conditions (for example, 1 versus 2 mol%; mean±s.e.m. ; Student’s t -test; P <0.05). Full size image To examine whether the labelling intensity with GST-PX is correlated with the PtdIns(3)P content, we compared liposomes containing different molar ratios (0.2–5%) of PtdIns(3)P. The labelling intensity, or the number of colloidal gold particles per μm 2 , increased roughly in proportion to the PtdIns(3)P content in the liposome ( Fig. 1b ). Although the absolute labelling intensity varied to some extent among different experimental sessions, the relative ratio of the labelling intensities in different membranes was reproducible. PtdIns(3)P distribution in yeast during logarithmic growth When PtdIns(3)P was labelled in the budding yeast Saccharomyces cerevisiae in log phase, intense labelling was observed in the cytoplasmic leaflet of the vacuolar membrane, which was represented as the protoplasmic face (PF) in the freeze-fracture replica ( Fig. 2a,b and Supplementary Fig. 1 ). Membranes of small cytoplasmic vesicles, which were probably endosome or prevacuolar compartments, were also labelled. On the other hand, virtually no labelling was observed in the luminal leaflet (represented as the exoplasmic face (EF)) of the vacuolar membrane or in other organellar membranes, including the plasma membrane, the nuclear membrane and the Golgi and mitochondrial membranes ( Fig. 2b,c and Supplementary Fig. 1a,b ). The abundance of PtdIns(3)P in the vacuolar membrane was consistent with previous results obtained by other methods employing a FYVE domain as a probe [11] , [19] . The PX domain of human p40 phox tagged with GFP was also targeted to the vacuolar membrane when expressed in yeast ( Supplementary Fig. 2 ). 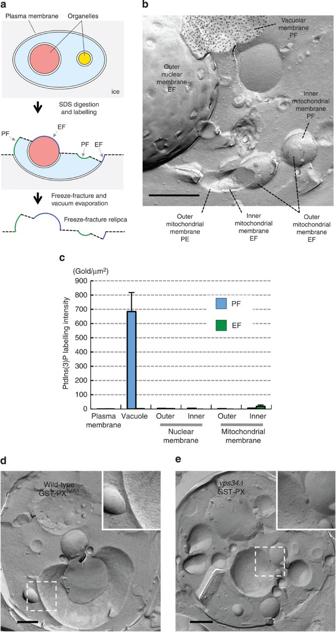Figure 2: PtdIns(3)P in yeast in log phase. (a) Outline of freeze-fracture EM. Replicas representing the outer (luminal) and inner (cytoplasmic) membrane leaflets are called the EF and the PF, respectively. Fracture planes passing through the cytoplasm and the extracellular space are shown by a dotted line. (b) QF-FRL in wild-type yeast in log phase. PtdIns(3)P was labelled with GFP-PX and marked with colloidal gold (10 nm). The vacuolar membrane PF was labelled intensely, whereas other organellar membranes did not exhibit significant labelling. Scale bar, 0.5 μm. (c) Quantification of the labelling intensity of PtdIns(3)P (mean±s.e.m.). The experiment was repeated three times and the number of colloidal gold particles per μm2was measured in more than ten randomly selected images. (d,e) Negative controls. Both wild-type yeast incubated with GST-PXR58A(d) andvps34Δyeast incubated with GST-PX (e) were virtually unlabelled. Scale bar, 0.5 μm. Figure 2: PtdIns(3)P in yeast in log phase. ( a ) Outline of freeze-fracture EM. Replicas representing the outer (luminal) and inner (cytoplasmic) membrane leaflets are called the EF and the PF, respectively. Fracture planes passing through the cytoplasm and the extracellular space are shown by a dotted line. ( b ) QF-FRL in wild-type yeast in log phase. PtdIns(3)P was labelled with GFP-PX and marked with colloidal gold (10 nm). The vacuolar membrane PF was labelled intensely, whereas other organellar membranes did not exhibit significant labelling. Scale bar, 0.5 μm. ( c ) Quantification of the labelling intensity of PtdIns(3)P (mean±s.e.m.). The experiment was repeated three times and the number of colloidal gold particles per μm 2 was measured in more than ten randomly selected images. ( d , e ) Negative controls. Both wild-type yeast incubated with GST-PX R58A ( d ) and vps34Δ yeast incubated with GST-PX ( e ) were virtually unlabelled. Scale bar, 0.5 μm. Full size image The labelling specificity of GST-PX in the cellular samples was verified by two control experiments. First, the freeze-fracture replica of wild-type yeast yielded no labelling when GST-PX was substituted with either GST-PX R58A or GST alone ( Fig. 2d ). Second, mutant yeasts lacking either Vps34p, the only PtdIns 3-kinase in yeast, or Vps15p, an indispensable component of PtdIns 3-kinase complexes, were not labelled with GST-PX ( Fig. 2e and Supplementary Fig. 1c ) [20] . Pretreatment of freeze-fracture replicas with proteinase K did not significantly change the labelling intensity with GST-PX, indicating that the labelling was neither derived from nor affected by proteins retained in the replica. PtdIns(3)P in autophagic membranes of yeast To observe the PtdIns(3)P distribution in autophagic membranes, yeast was cultured in nitrogen- and carbon-deficient S(-NC) medium for 2–5 h. This condition was used to induce autophagy in subsequent experiments because autophagosomes of relatively large sizes were observed most frequently [11] . Essentially the same result was obtained when autophagy was induced by nitrogen-deficient SD(-N) medium. In freeze-fracture EM, yeast autophagosomes were observed as spherical structures bounded by two smooth-surfaced layers [21] ( Fig. 3 ). The outer and inner membranes of the autophagosome can be unambiguously distinguished from the convexity/concavity of the structure as well as the membrane’s position at the near or far side of the double-layered membrane ( Fig. 3c ). Autophagic bodies in the vacuolar lumen were also observed as smooth-surfaced structures ( Fig. 4a,b ), consistent with the idea that autophagic bodies are derived from the inner autophagosomal membrane. Neither autophagosomes nor autophagic bodies were found in autophagy-deficient mutants, deleted with ATG2 , ATG3 , ATG5 , ATG7 , ATG8 , ATG9 , ATG12 , ATG16 , ATG18 , VPS15 or VPS34 . 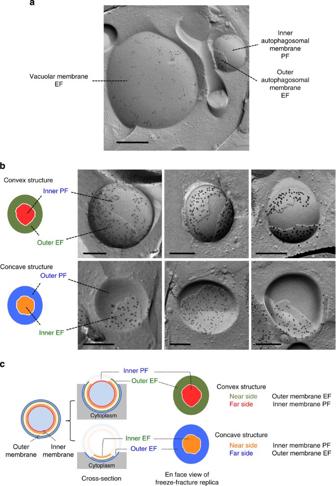Figure 3: PtdIns(3)P in yeast autophagosomes. (a) Wild-type yeast cultured in S(-NC) for 4 h. PtdIns(3)P was labelled intensely in the EF of autophagosomal membranes. A lower but still significant amount of labelling was also seen in the PF of autophagosome membranes as well as in the EF of the vacuolar membrane. Scale bar, 0.5 μm. (b) Autophagosomes in wild-type yeast cultured in S(-NC) for 4 h. The autophagosome was identified as a smooth-surfaced double-membrane structure, and seen in two different patterns, as shown in the diagrams inc. Upper panel: convex structures displaying the outer membrane EF and the inner membrane PF. Lower panel: concave structures displaying the outer membrane PF and the inner membrane EF. In both cases, PtdIns(3)P was labelled more intensely in the EF than in the PF. Scale bars, 0.2 μm. (c) Diagrams showing the membrane topologies of autophagosomes in freeze-fracture EM. Autophagosomes are observed as smooth-surfaced double-membrane structures in the cytoplasm. The outer and inner membranes can be distinguished based on the convexity or concavity of the structure, and whether the membrane appears as the near-side or far-side layer. Figure 3: PtdIns(3)P in yeast autophagosomes. ( a ) Wild-type yeast cultured in S(-NC) for 4 h. PtdIns(3)P was labelled intensely in the EF of autophagosomal membranes. A lower but still significant amount of labelling was also seen in the PF of autophagosome membranes as well as in the EF of the vacuolar membrane. Scale bar, 0.5 μm. ( b ) Autophagosomes in wild-type yeast cultured in S(-NC) for 4 h. The autophagosome was identified as a smooth-surfaced double-membrane structure, and seen in two different patterns, as shown in the diagrams in c . Upper panel: convex structures displaying the outer membrane EF and the inner membrane PF. Lower panel: concave structures displaying the outer membrane PF and the inner membrane EF. In both cases, PtdIns(3)P was labelled more intensely in the EF than in the PF. Scale bars, 0.2 μm. ( c ) Diagrams showing the membrane topologies of autophagosomes in freeze-fracture EM. Autophagosomes are observed as smooth-surfaced double-membrane structures in the cytoplasm. The outer and inner membranes can be distinguished based on the convexity or concavity of the structure, and whether the membrane appears as the near-side or far-side layer. 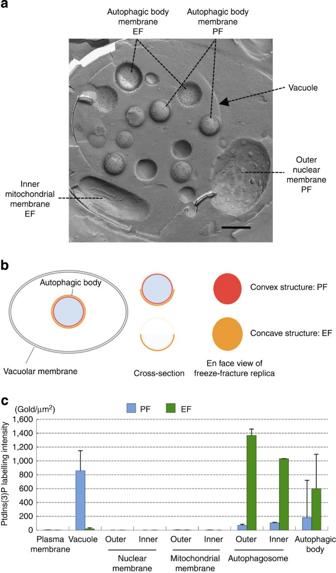Figure 4: PtdIns(3)P in yeast autophagic membranes. (a) Wild-type yeast cultured in S(-NC) for 4 h. PtdIns(3)P was labelled intensely in the EF of autophagic body membranes in the vacuolar lumen. A lower amount of labelling was also seen in the PF of autophagic body membranes. Scale bar, 0.5 μm. (b) Diagrams showing the membrane topologies of autophagic bodies in freeze-fracture EM. Autophagic bodies are observed as single-membrane structures in the vacuolar lumen. When an autophagic body appears as a convex structure the observed layer is the PF, whereas when it appears as a concave structure the observed layer is the EF. (c) Labelling intensity of PtdIns(3)P in wild-type yeast cultured in S(-NC) for 4 h (average±s.e.m.). PtdIns(3)P was found in both leaflets of the autophagosome and autophagic body membrane, and the labelling was much stronger in the EF than in the PF. In the vacuolar membrane, significant labelling was found in the EF, albeit at much lower levels than in the PF. The experiment was repeated three times, and the number of colloidal gold particles per μm2was measured in more than ten randomly selected images. Full size image Figure 4: PtdIns(3)P in yeast autophagic membranes. ( a ) Wild-type yeast cultured in S(-NC) for 4 h. PtdIns(3)P was labelled intensely in the EF of autophagic body membranes in the vacuolar lumen. A lower amount of labelling was also seen in the PF of autophagic body membranes. Scale bar, 0.5 μm. ( b ) Diagrams showing the membrane topologies of autophagic bodies in freeze-fracture EM. Autophagic bodies are observed as single-membrane structures in the vacuolar lumen. When an autophagic body appears as a convex structure the observed layer is the PF, whereas when it appears as a concave structure the observed layer is the EF. ( c ) Labelling intensity of PtdIns(3)P in wild-type yeast cultured in S(-NC) for 4 h (average±s.e.m.). PtdIns(3)P was found in both leaflets of the autophagosome and autophagic body membrane, and the labelling was much stronger in the EF than in the PF. In the vacuolar membrane, significant labelling was found in the EF, albeit at much lower levels than in the PF. The experiment was repeated three times, and the number of colloidal gold particles per μm 2 was measured in more than ten randomly selected images. Full size image Surprisingly, PtdIns(3)P in yeast autophagosomal membranes was labelled in both the PF and the EF (representing the cytoplasmic and luminal leaflet, respectively); moreover, the labelling intensity was significantly greater in the EF than in the PF of both the inner and outer autophagosomal membranes ( Figs 3b and 4c ). Using the labelling intensity in the liposome replica as a scale ( Fig. 1b ), we estimated the PtdIns(3)P content in the luminal and cytoplasmic leaflet to be >5% and <1%, respectively. PtdIns(3)P was also labelled intensely in the autophagic body membranes, again showing the luminal leaflet-dominant asymmetry ( Fig. 4a,c ). This asymmetry was different from that of the internal vesicle membrane of the multivesicular body, in which PtdIns(3)P is thought to exist only in the cytoplasmic leaflet [22] . In cells undergoing autophagy, the EF of the vacuolar membrane also exhibited a small increase in PtdIns(3)P labelling ( Figs 3a and 4c ), probably caused by fusion of the outer autophagosomal membrane to the vacuolar membrane. However, considering that many autophagosomes fuse with a single vacuole, the observed increase of PtdIns(3)P in the vacuolar membrane was far lower than the amount predicted to be added by autophagosome fusion. This finding suggested that efficient mechanisms must exist to remove PtdIns(3)P on the luminal surface of the vacuolar membrane. Degradation by phosphatases and/or lipases is a possibility, but the PtdIns(3)P labelling intensity did not increase in atg15Δ , arguing against the involvement of this putative lipase [23] . Alternatively, membranes enriched with PtdIns(3)P in the luminal leaflet may be retrieved from the vacuole. Indeed, deletion of VAC7 , which suppresses PtdIns(3)P 5-kinase activity [24] and division of vacuoles [25] , increased PtdIns(3)P in the EF of the vacuolar membrane. However, the increase of PtdIns(3)P in the luminal leaflet of the vacuolar membrane was relatively small in vac7Δ , indicating that other mechanisms, involving other phosphatases and lipases or flipping of PtdIns(3)P to the cytoplasmic leaflet, are likely to exist. Phosphoinositides were labelled specifically in ultrathin cryosections [19] . By using GST-PX, this method yielded labelling in vacuoles and small cytoplasmic vesicles of wild-type yeast ( Supplementary Fig. 3 ). The labelling was dependent on PtdIns(3)P, because it was not observed when cells were labelled with GST-PX R58A or in vps34Δ cells. However, labelling in cryosections was scarcely observed on the cytoplasmic side of the vacuolar membrane, where PtdIns(3)P should be present [11] , whereas abundant labelling was observed on the luminal side of the membrane ( Supplementary Fig. 3 ). The paucity of labelling on the cytoplasmic side of the vacuolar membrane may be due to the inability of aldehydes to fix lipids and/or poor penetration of the GST-PX probe into the cytoplasmic matrix. This result indicated that cryosectioning would not be an effective method for localizing PtdIns(3)P in autophagosomal membranes. PtdIns(3)P in mammalian autophagosomal membranes We next examined how PtdIns(3)P distributes in mammalian autophagosomal membranes. As autophagosomes induced by starvation or other conventional means have been observed only infrequently by freeze-fracture EM, two methods were used to increase the chance of encounter. In the first method, Huh7 cells expressing GFP-LC3 were treated with Torin1 in the presence of bafilomycin A1, to increase the number of autophagosomes by suppressing autophagosome–lysosome fusion [26] . Although the effects of bafilomycin A1 vary depending on experimental conditions [27] , treatment with 0.25 μM Torin1 and 0.4 μM bafilomycin A1 for 1 h increased GFP-LC3-positive, Lamp1-negative autophagosomes in Huh7 cells ( Supplementary Fig. 4a ), and this increase was also confirmed by conventional EM ( Supplementary Fig. 4b ). In freeze-fracture EM, autophagosomes were identified by their typical morphology (that is, double-membrane structure with few intramembrane particles (IMPs)) [28] and the presence of GFP-LC3 ( Fig. 5a and Supplementary Fig. 4c ). In autophagosomal membranes, both PtdIns(3)P and GFP-LC3 were labelled predominantly in the PF (that is, the cytoplasmic leaflet; Fig. 5a,c and Supplementary Fig. 4c ). Although a few colloidal gold particles representing PtdIns(3)P were also observed in the EF, they were always found in regions where the EF of one autophagosomal membrane abutted directly against the PF of another autophagosomal membrane ( Fig. 5a and Supplementary Fig. 4c ). Considering that the arm distance from the target molecule to the centre of colloidal gold is ~16 nm (ref. 16 ), it is likely to be that labelling on the edge of the EF actually represented PtdIns(3)P in the PF of an adjacent autophagosomal membrane. 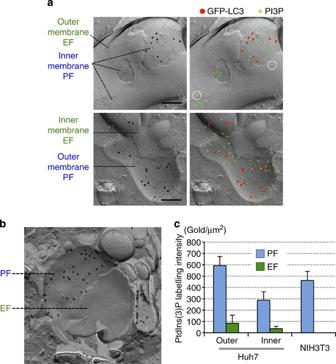Figure 5: PtdIns(3)P in mammalian autophagosomal membrane. (a) Huh7 cells expressing GFP-LC3 treated with 0.25 μM Torin1 and 0.4 μM bafilomycin A1 for 1 h. The autophagosome was identified as the IMP-poor double-membrane structure labelled with anti-GFP antibody (large gold, 10 nm). Both PtdIns(3)P (small gold, 6 nm) and GFP-LC3 were seen exclusively in the PF in both convex and concave structures. The small and large gold particles are shown as green and red dots, respectively, in the figures at right. Scale bars, 0.1 μm. Figures displaying wider areas, as well as additional examples, are presented inSupplementary Fig. 4c. (b) NIH3T3 cells expressing Atg4C78Awere incubated in Earle’s balanced salt solution for 1 h. The isolation membrane was observed as parallel membranes with few IMPs. PtdIns(3)P was labelled only in the PF. Scale bar, 0.1 μm. Other examples are presented inSupplementary Fig. 5. (c) Labelling density of PtdIns(3)P in mammalian autophagosomal membrane (mean±s.e.m.). The experiment was repeated three times and the number of colloidal gold particles per μm2was measured in more than ten randomly selected images. Some labelling was observed in the EF but the majority of gold particles in the EF occurred near the EF-PF boundary (white circles; seeSupplementary Fig. 6cfor more examples), suggesting that many of them actually represent PtdIns(3)P in the PF. Figure 5: PtdIns(3)P in mammalian autophagosomal membrane. ( a ) Huh7 cells expressing GFP-LC3 treated with 0.25 μM Torin1 and 0.4 μM bafilomycin A1 for 1 h. The autophagosome was identified as the IMP-poor double-membrane structure labelled with anti-GFP antibody (large gold, 10 nm). Both PtdIns(3)P (small gold, 6 nm) and GFP-LC3 were seen exclusively in the PF in both convex and concave structures. The small and large gold particles are shown as green and red dots, respectively, in the figures at right. Scale bars, 0.1 μm. Figures displaying wider areas, as well as additional examples, are presented in Supplementary Fig. 4c . ( b ) NIH3T3 cells expressing Atg4 C78A were incubated in Earle’s balanced salt solution for 1 h. The isolation membrane was observed as parallel membranes with few IMPs. PtdIns(3)P was labelled only in the PF. Scale bar, 0.1 μm. Other examples are presented in Supplementary Fig. 5 . ( c ) Labelling density of PtdIns(3)P in mammalian autophagosomal membrane (mean±s.e.m.). The experiment was repeated three times and the number of colloidal gold particles per μm 2 was measured in more than ten randomly selected images. Some labelling was observed in the EF but the majority of gold particles in the EF occurred near the EF-PF boundary (white circles; see Supplementary Fig. 6c for more examples), suggesting that many of them actually represent PtdIns(3)P in the PF. Full size image In the second manipulation intended to increase the rate of observation of mammalian autophagosomes, we used NIH3T3 cells overexpressing a dominant-negative Atg4 protein, Atg4 C78A . Atg4 C78A perturbs lipidation of LC3 and induces abundant unclosed autophagosomes in starved cells [29] . The autophagosomes thus generated do not harbour LC3, but are instead observed as IMP-poor double-layered membranes. PtdIns(3)P was labelled exclusively in the PF of those autophagosomal membranes ( Fig. 5b,c and Supplementary Fig. 5 ). Effect of PtdIns(3)P phosphatase depletion The results described above revealed that autophagosomal membranes in yeast and mammalian cells differ significantly with regard to PtdIns(3)P distribution. The exclusive presence of PtdIns(3)P in the cytoplasmic leaflet of mammalian autophagosome membranes is consistent with the current understanding that PtdIns(3)P is generated by PtdIns 3-kinase acting on phosphatidylinositol in existing organelle membranes [5] , [6] , [7] , [8] . However, in this study we observed the opposite asymmetry in yeast autophagosomal membranes (that is, luminal>cytoplasmic), which cannot be explained by the same mechanism. Therefore, we next hypothesized that when yeast isolation membranes are initially formed, they harbour equivalent amounts of PtdIns(3)P in both leaflets; subsequently, the observed asymmetry in the autophagosomal membrane is generated through unilateral hydrolysis of PtdIns(3)P by cytoplasmic phosphatases ( Fig. 6c ). 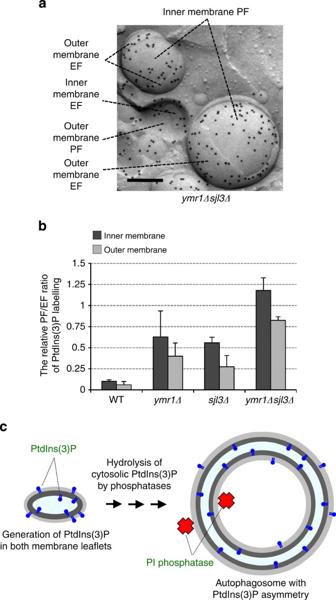Figure 6:PtdIns(3)P inymr1Δsjl3Δ. (a)ymr1Δsjl3Δcells cultured in S(-NC) for 4 h. PtdIns(3)P was labelled in comparable densities in PF and EF of autophagosomal membranes. Scale bar, 0.2 μm. (b) The PF/EF ratio of the PtdIns(3)P labelling density in autophagosomal membrane (mean±s.e.m.). The ratio was small (that is, PF≅EF) inymr1Δsjl3Δ. The experiment was repeated three times and the number of colloidal gold particles per μm2was measured in more than ten randomly selected images. (c) A hypothetical mechanism to generate the PtdIns(3)P asymmetry in yeast autophagic membranes. PtdIns(3)P is formed not only in the cytoplasmic leaflet but also in the luminal leaflet of the isolation membrane and/or the autophagosome by an unknown mechanism(s). PtdIns(3)P in the cytoplasmic leaflet, but not that in the luminal leaflet, is hydrolysed by phosphatases, resulting in the observed PtdIns(3)P asymmetry. Figure 6: PtdIns(3)P in ymr1Δsjl3Δ . ( a ) ymr1Δsjl3Δ cells cultured in S(-NC) for 4 h. PtdIns(3)P was labelled in comparable densities in PF and EF of autophagosomal membranes. Scale bar, 0.2 μm. ( b ) The PF/EF ratio of the PtdIns(3)P labelling density in autophagosomal membrane (mean±s.e.m.). The ratio was small (that is, PF ≅EF) in ymr1Δsjl3Δ . The experiment was repeated three times and the number of colloidal gold particles per μm 2 was measured in more than ten randomly selected images. ( c ) A hypothetical mechanism to generate the PtdIns(3)P asymmetry in yeast autophagic membranes. PtdIns(3)P is formed not only in the cytoplasmic leaflet but also in the luminal leaflet of the isolation membrane and/or the autophagosome by an unknown mechanism(s). PtdIns(3)P in the cytoplasmic leaflet, but not that in the luminal leaflet, is hydrolysed by phosphatases, resulting in the observed PtdIns(3)P asymmetry. Full size image To test this hypothesis, we examined yeasts lacking a myotubularin-related phosphatase Ymr1p [30] , a synaptojanin-like phosphatase Sjl3p [31] , or both proteins. As described above, the relative labelling intensity of PtdIns(3)P in the two leaflets, expressed as the PF/EF ratio, was very low in wild-type cells ( Figs 4c and 6b ). By contrast, ymr1Δ and sjl3Δ cells exhibited a higher PF/EF ratio than wild-type cells, but the PtdIns(3)P asymmetry remained. Only in ymr1Δsjl3Δ cells did the labelling intensity in the PF and EF become almost comparable, resulting in a PF/EF ratio close to 1 ( Fig. 6a,b ). These results were consistent with our hypothesis that the asymmetrical PtdIns(3)P distribution in yeast autophagosomal membranes is a result of hydrolysis by Ymr1p and Sjl3p ( Fig. 6c ). It is not clear how PtdIns(3)P can remain abundant in the cytoplasmic leaflet of mammalian autophagosomal membranes despite the presence of cytoplasmic phosphatases [32] . We speculate that in mammals the activity of phosphatases may be low relative to the rate of PtdIns(3)P synthesis, or that a majority of PtdIns(3)P molecules may be bound by PtdIns(3)P-binding proteins and therefore be protected from hydrolysis. In accordance with a recent report [33] , autophagic bodies were scarce in ymr1Δsjl3Δ cells ( Supplementary Fig. 6a ). Consistent with this, the processing of aminopeptidase I was comparable in wild-type, ymr1Δ and sjl3Δ cells, but not in ymr1Δsjl3Δ cells ( Supplementary Fig. 6b ). On the other hand, conjugation of Atg8 to phosphatidylethanolamine did occur in ymr1Δsjl3Δ cells ( Supplementary Fig. 6c ), suggesting that the autophagic process may begin normally but be blocked at a later stage. In this context, it was notable that autophagosomes in ymr1Δsjl3Δ cells often exhibited distorted shapes with aberrant constrictions and creases ( Supplementary Fig. 7 ). This result suggested that excessive PtdIns(3)P in the cytoplasmic membrane leaflet may induce a structural abnormality in the autophagosome, disturbing its closure and fusion with the vacuole [33] . The most important finding of this study is the presence of PtdIns(3)P in the luminal leaflet of the yeast autophagosomal membrane. Luminal (or extracellular) PtdIns(3)P has been reported to exist in the endoplasmic reticulum membrane of malaria parasite Plasmodium falciparum [34] and in the plasma membranes of plant and mammalian cells [35] , but the mechanism of generation is not known. We envision several possible explanations for our finding. First, PtdIns(3)P generated in the cytoplasmic side of the membrane may flip to the luminal side. Although it is not clear whether PtdIns(3)P can translocate across the membrane, previous work has shown that other lipids, including phosphatidylinositol [36] and the oligosaccharide diphosphate dolichol [37] , can do so. Importantly in this regard, the latter lipid has a much bulkier hydrophilic head portion than PtdIns(3)P. Although the paucity of IMPs suggests that transmembrane proteins are not abundant in the autophagosomal membrane, some flippase may nonetheless be present [38] . Second, random mixing of the membrane lipids of the luminal and cytoplasmic leaflets may occur in a non-bilayer structure. EM studies have revealed that the yeast isolation membrane is thinner than other membranes and is seldom seen as a canonical bilayer structure [39] . This may be because the isolation membrane assumes a non-bilayer structure, either locally or transiently, due to enrichment of a hexagonal (H II )-lipid, phosphatidylethanolamine [40] . Third, some yeast organelle membranes may contain PtdIns(3)P in the luminal leaflet, as in other species [34] , [35] and these membranes may contribute to formation of the isolation membrane. Fourth, de novo membrane assembly may contribute to formation of the yeast isolation membrane [41] and PtdIns 3-kinase already present in the nascent lumen may generate PtdIns(3)P in the luminal leaflet. These possibilities are not mutually exclusive with each other and they should all be addressed in future studies. Whatever the mechanism may be, the observed difference in PtdIns(3)P distribution suggests that autophagy involves different processes in yeast and mammals. This is surprising in light of the general conservation of autophagy-related molecules [42] . Nonetheless, several important differences between autophagic mechanisms in yeast and mammals have already been elucidated: isolation membranes in yeast form at a single PAS adjacent to the vacuole, whereas those in mammals are generated at multiple sites [43] ; yeast Atg14 is targeted to the PAS, whereas mammalian Atg14L is recruited to the endoplasmic reticulum [44] , [45] ; and as revealed by freeze-fracture EM, autophagosomes are invariably spherical in yeast, whereas they assume heterogeneous shapes in mammals (this study, compare Fig. 3b and Fig. 5a.b ). Furthermore, yeast Atg27p, a transmembrane protein that contains a PtdIns(3)P-binding sequence in its luminal region, has no orthologue in mammals [46] . Presumably, these differences evolved in response to divergent demands for autophagy between yeast and mammalian cells. Elucidating the molecular mechanism by which PtdIns(3)P is generated in the luminal membrane leaflet will be critical to a more detailed understanding of autophagosome formation. Probes Complementary DNA generated by RT–PCR of human THP-1 cell total RNA was used as a template to clone the PX domain of p40 Phox (primers 5′-GCTGTGGCCCAGCAGCTGCGGGCCGAG-3′ and 5′-TCACCGGCGGATGGCCTGGGGCACCTG-3′) and the FYVE domain of FENS-1 (primers 5′-AGCAGAGAAGAGGCTCCTCAGTGGTTGGA-3′ and 5′-TTAGAAGTCCGATCTTCATCTTTGATGGAGTCG-3′) [17] . Recombinant GST-PX and its mutant GST-PX R58A , which lacks PtdIns(3)P-binding capacity [47] , were produced in Escherichia coli and affinity purified on a glutathione-agarose column [16] . Rabbit anti-Atg8 antibody was described previously [48] . Rabbit anti-GFP antibody was kindly provided by Dr Masahiko Watanabe (Hokkaido University) [49] . Other primary antibodies were rabbit anti-GST (Bethyl, A190-122A), mouse anti-GST (BioLegend, 640802) and mouse anti-Lamp1 (Developmental Studies Hybridoma Bank, H4A3). Colloidal gold particles that were conjugated with either protein A (The University Medical Center Utrecht, PAG 10 nm), goat anti-rabbit IgG (BBInternational, EM.GAR10) or donkey anti-mouse IgG (Jackson ImmunoResearch, 715-195-150) were used. Liposomes Phosphatidylcholine (Avanti) and the protonated forms of phosphoinositides (Cell Signals) were dissolved in chloroform at defined molar ratios, dried in dry nitrogen gas and vortexed with an aqueous buffer to make liposomes. The liposome solution was pushed through a Mini-extruder (Avanti) equipped with a polycarbonate membrane filter (pore size: 0.1 or 0.2 μm) to make unilamellar vesicles. Yeast All yeast strains used in this study are based on the parent strain SEY6210 ( Table 1 ). Generation of deletion mutants was performed by a PCR-based method using pFA6a plasmids as templates [50] . To induce autophagy, cells cultured in YPD medium (1% yeast extract, 2% polypeptone and 2% dextrose) were washed with water and incubated for 3–5 h at 30 °C in nitrogen- and carbon-depleted medium S (-NC) (0.17% yeast nitrogen base without amino acids and ammonium sulphate (Becton Dickinson)) or in nitrogen-depleted medium SD(-N) (0.17% yeast nitrogen base without amino acids and ammonium sulphate (Becton Dickinson) and 2% dextrose). Both S (-NC) and SD(-N) media were supplemented with 1 mM phenylmethyl sulphonyl fluoride (Sigma). Table 1 Strains used in this study. Full size table Mammalian cells Huh7 cells stably expressing GFP-LC3 were generated by transfection of a plasmid vector and selection using G418 (ref. 51 ). A stable NIH3T3 cell line expressing Atg4B C74A (ref. 29 ) was kindly provided by Dr Tamotsu Yoshimori (Osaka University). The cells were cultured in Dulbecco's modified Eagle's medium supplemented with 10% FCS and antibiotics, and kept in a humidified atmosphere containing 5% CO 2 . To observe autophagic membranes, Huh7 cells were treated with 0.25 μM Torin1 and 0.2 μM bafilomycin A1 in normal medium for 1–2 h, and NIH3T3 cells were incubated in Earle’s balanced salt solution (Invitrogen) for 1 h. Western blotting To prepare yeast cell lysates, cells were vortexed with zirconia/silica beads in 10% trichloroacetic acid and 1 mM phenylmethyl sulphonyl fluoride. The precipitated sample was dissolved in SDS sample buffer (2% SDS, 10% glycerol, 60 mM Tris–HCl, pH 6.8), and supernatant after centrifugation was loaded for SDS–PAGE, electrotransferred to polyvinylidene difluoride membrane and subjected to western blotting. For investigations of Atg8–phosphatidylethanolamine conjugation, 6 M urea was added to the acrylamide gel [39] . Full blots are shown in Supplementary Fig. 8 . Immunofluorescence microscopy Huh7 cells expressing GFP-LC3 cultured on glass coverslips were fixed with a mixture of 0.025% glutaraldehyde and 3% formaldehyde in 0.1 M sodium phosphate buffer (pH 7.4) for 15 min, permeabilized with 0.01% digitonin in PBS for 30 min and treated with 5% normal goat serum in PBS for 10 min. The cells were then labelled for with anti-Lamp1 antibody (5 μg ml −1 ) and confocal images were collected with a Zeiss PASCAL confocal system mounted on a Zeiss Axioplan2 microscope equipped with a × 63 NA1.4 Apochromat objective lens. All fluorescence images show a single focal z section. Structured illumination microscopy Yeast cells expressing GFP alone or GFP-PX were incubated with FM4-64 (Biotium) to label the vacuolar membrane, and then observed in log phase or after autophagic induction under a Axiovert microscope (Zeiss) using a × 63 NA1.4 Apochromat objective lens. Optical sections were obtained using an Apotome structured illumination microscopic system (Zeiss). Quick-freezing and freeze-fracture replica labelling method A gold EM grid (200 mesh) impregnated with yeast cells or liposome pellets was sandwiched between two flat aluminum discs (Engineering Office M. Wohlwend). Mammalian cells were treated in two different ways: some were detached from the substrate by a brief treatment with trypsin and EDTA, and processed similarly to yeast; the others were cultured on a 20-μm-thick gold foil and inserted between the flat aluminum disc and another disk with a 0.3-mm indentation [52] . The sample assemblies were frozen using an HPM 010 high-pressure freezing machine (Leica) according to the manufacturer’s instructions. The time required for freezing was ~10 ms, which should be sufficiently fast to preserve PtdIns(3)P distribution in situ . For freeze fracture, the specimens were transferred to the cold stage of a Balzers BAF 400 apparatus and fractured at −130 to −115 °C under a vacuum of~1 × 10 −6 mbar. Replicas were made by electron-beam evaporation in three steps: carbon (C) (2–5 nm in thickness) at an angle of 90° to the specimen surface, platinum–carbon (1–2 nm) at an angle of 45° and C (10–20 nm) at an angle of 0° (ref. 14 ). The thickness of the deposition was adjusted by referring to a crystal thickness monitor. Thawed replicas were treated with 2.5% SDS in 0.1 M Tris–HCl (pH 7.4) at 60 °C overnight. To remove the cell wall, yeast replicas were digested with 1 mg ml −1 Zymolyase 20T in PBS containing 0.1% Triton X-100, 1% BSA and a protease inhibitor cocktail (Nacalai Tesque) for 2 h at 37 °C. After a further treatment in 2.5% SDS, the replicas were stored in buffered 50% glycerol at −20 °C until use. Replica labelling Freeze-fracture replicas were washed with PBS containing 0.1% Triton X-100 (PBST), blocked with 3% BSA in PBST and incubated at 4 °C overnight with GST-PX or GST-PX R58A (10 ng ml −1 ) in PBS containing 1% BSA. The samples were subsequently treated with rabbit anti-GST antibody (10 μg ml −1 ) followed by colloidal gold (10 nm)-conjugated protein A (PAG10; 1:60 dilution of the supplied solution), both for 30 min at 37 °C in 1% BSA in PBST. For double labelling of PI3P and GFP-LC3 in mammalian cells, the secondary incubation was performed using a combination of mouse anti-GST antibody (10 μg ml −1 ) and rabbit anti-GFP antibody, and the tertiary incubation used a combination of colloidal gold (6 nm)-conjugated donkey anti-mouse IgG (1:60 dilution of the supplied solution) and colloidal gold (10 nm)-conjugated goat anti-rabbit antibody (1:30 dilution of the supplied solution). After each incubation, replicas were washed extensively with 0.1% BSA in PBST. After brief rinses with distilled water, replicas were picked up on Formvar-coated EM grids and observed with a JEOL JEM-1011 EM operated at 100 kV. Digital images were captured using a charge-coupled device camera (Gatan) and subjected to further analysis. Labelling of ultrathin cryosections Yeast cells were fixed with a mixture of 0.05% glutaraldehyde and 4% paraformaldehyde in 0.1 M PHEM (20 mM PIPES, 50 mM HEPES, 20 mM EGTA, 4 mM MgCl 2 , pH 6.9) for 3 h, treated with 1% sodium periodate in 0.1 M PHEM for 1 h and infiltrated with 2.3 M sucrose overnight before freezing [53] . Ultrathin cryosections were blocked with 3% BSA in PBS, and incubated at 4 °C overnight with GST-PX or GST-PX R58A (10 ng ml −1 ) in PBS containing 1% BSA. Sections were then treated with rabbit anti-GST antibody (10 μg ml −1 ) followed by PAG10, both for 30 min at 37 °C in 1% BSA in PBS. After treatment with 2% glutaraldehyde, the sections were infiltrated with a mixture of 2% methylcellulose and 0.5% uranyl acetate, dried and observed by transmission EM. Conventional EM Yeast cells were fixed with a mixture of 1% glutaraldehyde and 0.2% paraformaldehyde in 40 mM potassium phosphate (pH 7.0), then with 2% potassium permanganate, dehydrated and embedded in Spurr’s low-viscosity resin [54] . Ultrathin sections were observed with a transmission EM after counterstaining with uranyl acetate and lead citrate. Statistical analysis EM images obtained from more than three independent experiments were used for the analysis. The number of colloidal gold particles was counted manually, and areas were measured using ImageJ (NIH). The labelling density in the selected structure was calculated by dividing the number of colloidal gold particles by the area. For each structure, the labelling density was measured in more than ten different micrographs that were taken randomly. Statistical differences between samples were tested using Student’s t -test. How to cite this article : Cheng, J. et al . Yeast and mammalian autophagosomes exhibit distinct phosphatidylinositol 3-phosphate asymmetries. Nat. Commun. 5:3207 doi: 10.1038/ncomms4207 (2014).